Analysis of protein-coding mutations in hiPSCs and their possible role during somatic cell reprogramming Recent studies indicate that human-induced pluripotent stem cells contain genomic structural variations and point mutations in coding regions. However, these studies have focused on fibroblast-derived human induced pluripotent stem cells, and it is currently unknown whether the use of alternative somatic cell sources with varying reprogramming efficiencies would result in different levels of genetic alterations. Here we characterize the genomic integrity of eight human induced pluripotent stem cell lines derived from five different non-fibroblast somatic cell types. We show that protein-coding mutations are a general feature of the human induced pluripotent stem cell state and are independent of somatic cell source. Furthermore, we analyse a total of 17 point mutations found in human induced pluripotent stem cells and demonstrate that they do not generally facilitate the acquisition of pluripotency and thus are not likely to provide a selective advantage for reprogramming. The induction of pluripotency in human somatic cells by defined transcription factors represents a breakthrough in regenerative medicine [1] , [2] , [3] , [4] , [5] . The generation of patient-specific human induced pluripotent stem cells (hiPSCs) and their autologous cell derivatives would help to overcome the problems of immune rejection and tissue availability. However, the applications of cell therapies in human patients are subject to very stringent safety requirements, and there is a general concern in the field about the safety of hiPSCs. Successful generation of hiPSCs depends on the complete reprogramming of the somatic epigenome to a pluripotent state while the genome remains unchanged. Although initial reports demonstrated that human embryonic stem cells (hESCs) and hiPSCs were very similar, recent reports have uncovered striking genetic and epigenetic differences between these two pluripotent cell types [6] , [7] , [8] , [9] , [10] , [11] . It has been shown that hiPSCs display protein-coding mutations, large-scale genomic rearrangements, persistent epigenetic marks from the somatic cell type of origin and aberrant methylation patterns [6] , [9] , [11] . These findings indicated that hiPSCs contain genomic defects that could preclude their use in stem cell therapies. However, most of these studies focused on fibroblast-derived hiPSCs, and a more comprehensive analysis is essential to determine whether there are specific somatic cell types that may reprogram into hiPSCs with fewer (or perhaps none) of these aberrations. Additionally, it is unclear whether the protein-coding mutations found in hiPSCs provide any functional advantage and, thus, are selected for during the process of reprogramming. In this work, we characterize at single-nucleotide resolution the genomic integrity of eight hiPSC lines derived from five different non-fibroblast somatic cell types with varied reprogramming efficiencies. Moreover, we functionally characterize the role of 17 point mutations found in hiPSCs for their ability to increase reprogramming efficiency. We demonstrate that the majority of these mutations do not favour the reprogramming process and suggest that most of them originated randomly or were initially present in the somatic population of origin. Our observations of the genetic abnormalities of hiPSCs will contribute to a deeper understanding of the reprogramming process. hiPSC lines from varied cell types contain protein-coding mutations We previously sequenced the protein-coding regions of 22 fibroblast-derived hiPSC lines and discovered that the hiPSCs analysed carried between 2 and 14 point mutations in protein-coding regions [6] . In this study, we sought to determine whether low reprogramming efficiency (and therefore a potentially higher level of selection pressure that could allow the fixation of advantageous mutations) or cell type of origin (as fibroblasts could possess a higher somatic mutation rate than other cell types) could contribute to the overall reprogramming-associated mutational load. To this end, we performed targeted exome sequencing on eight non-fibroblast-derived hiPSC lines and their five somatic cell types of origin using an in-solution hybridization capture method ( Supplementary Table S1 ). Somatic mutations in each hiPSC line were identified via pairwise comparison with the matched somatic cell of origin and independently confirmed with capillary Sanger sequencing. 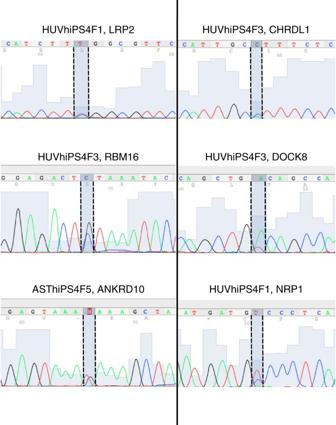Figure 1: Mutated alleles are expressed in hiPSC lines. Sanger chromatograms showing the results of RNA Sequencing analysis performed on the indicated genes found mutated in the indicated hiPSC lines. Dashed lines highlight the point-mutated nucleotide. Note the expression of both reference and mutated alleles in all cases analyzed. We identified a total of 40 point mutations throughout all the hiPSC lines analysed, leading to an average of five coding mutations per line ( Table 1 ). As we identified ~89% of expected total single-nucleotide polymorphisms at high sequencing depth in protein-coding regions, this led to a projection of 45 total mutations in protein-coding regions, or ~6 coding mutations per cell line. The levels of mutational load from each individual somatic cell type were statistically indistinguishable, and within the range previously observed for fibroblast-derived hiPSC lines [6] ( Table 1 ). These results indicate that hiPSC-associated mutations cannot be avoided by using younger or potentially more genetically protected somatic cell sources as progenitor cells. Moreover, we determined that reprogramming efficiency, which varies between 0.001 to 3% for these cell types, did not seem to have a measurable effect on the hiPSC mutational load. Thus, reprogramming-associated point mutations appear to be a general feature of hiPSCs. Table 1 List of protein-coding mutations in hiPSC lines. Full size table We next investigated whether mutations in hiPSCs were either enriched or depleted in protein-coding regions. 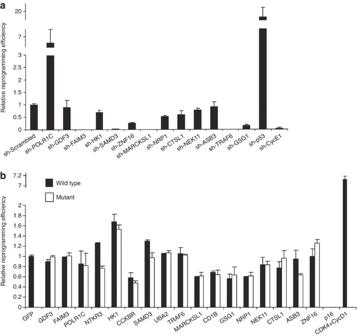Figure 2: Evaluation of the functional effect of hiPSC mutations on reprogramming efficiency. (a,b) Human BJ fibroblasts were infected with retroviruses encoding OSKC, and either lentiviruses encoding shRNAs against the indicated proteins (a) or retroviruses encoding the wild type or mutated proteins (b). Relative reprogramming efficiencies (evaluated as percentage of Nanog+colonies) are shown as fold change normalized to the averaged efficiency observed in (a) pLVTHM or (b) pMX–GFP-infected fibroblasts. Ina, lentiviruses encoding shRNAs againstCycE1orp53were used as controls of reduced or increased reprogramming efficiency, respectively. Inb, retroviruses encodingp16or the pair CDK4/CycD1 were used as controls of reduced or increased reprogramming efficiency, respectively. Fora, 20,000 infected cells were plated when shRNAs againstPOLR1Candp53were used, and 70,000 infected cells were plated under all other conditions. Forb, a total of 25,000 infected cells were plated under all conditions. Two independent experiments with two biological replicates were carried out. All error bars depict the s.d. To this end, we examined additional non-coding regions captured in our sequencing analysis, and found a similar mutation rate per base pair analysed for both coding and non-coding regions ( Table 2 ). We also investigated whether point mutations in hiPSCs tended to occur in active/ubiquitous or silent/tissue-specific genes. Among a total of 132 mutated genes (from this study and ref. 6 ) annotated in the TiGER Database [12] , 37% of these genes showed tissue-specific expression, which is very similar to the overall level of tissue specificity observed in the genes annotated in the database (34%; P =0.4975), indicating that mutations are not preferentially occurring in silent genes. We additionally checked for any potential enrichment of mutations in active or inactive transcriptional regions of the genome [13] . We found that mutations were not significantly enriched in the active or inactive chromatin regions of fibroblasts ( P =0.79), hESCs ( P =0.29) or hiPSCs ( P =0.07). Furthermore, only one gene ( NTRK3 ) was found mutated in more than one independent hiPSC line, and mutated genes did not cluster in a specific functional pathway (ref. 6 and results herein). These combined findings suggest that mutations in hiPSCs are spread throughout both transcriptionally active and silent regions of the genome. Table 2 List of candidate non-coding mutations in hiPSC lines. Full size table hiPSC-point mutations do not favour the process of reprogramming We previously showed that at least half of reprogramming-associated point mutations pre-exist in starting somatic cell populations at low frequency [6] . This leads to a hypothesis that a sub-population of somatic cells carrying certain mutations could be primed for reprogramming, which would be consistent with the elite model for reprogramming [14] . To investigate the functional potential of these mutations during reprogramming, we first assessed whether mutated alleles were expressed in the hiPSC lines. We isolated RNA from three hiPSC lines, reverse-transcribed it into cDNA and sequenced a total of six transcripts of randomly selected genes found mutated in these hiPSC lines. We detected heterozygous expression of both mutant (mut) and wild-type(wt) alleles in all cases ( Fig. 1 ), indicating that mutated transcripts are expressed in hiPSCs. Figure 1: Mutated alleles are expressed in hiPSC lines. Sanger chromatograms showing the results of RNA Sequencing analysis performed on the indicated genes found mutated in the indicated hiPSC lines. Dashed lines highlight the point-mutated nucleotide. Note the expression of both reference and mutated alleles in all cases analyzed. Full size image We next sought to determine whether reprogramming-associated mutations could contribute functionally in facilitating the acquisition of pluripotency during reprogramming. From a total of 164 different genes found mutated in hiPSC lines (ref. 6 and this study), we assayed the function of 17 candidate genes and their mutated forms during reprogramming ( Supplementary Table S2 ). These candidate genes were selected based on the likelihood of the mutation to change protein function, the mutation type (only non-synonymous mutations were analysed) and whether the gene was known to be related to the maintenance and/or acquisition of pluripotency [6] ( Table 1 ; Supplementary Fig. S1 ; Supplementary Table S2 ). We also analysed the expression of these 17 genes in BJ fibroblasts, human umbilical vein endothelial cells (HUVEC), hESC and hiPSC lines to ensure gene expression in at least one of the somatic cell types used in this work ( Supplementary Fig. S2 ). Owing to the difficulty in predicting the functional consequences of each specific mutation, we first performed ‘loss-of-function’ reprogramming experiments to mimic a possible diminished activity or protein instability of the mutated form. To this end, we designed a panel of lentiviruses encoding short hairpin RNAs (shRNAs) against the selected genes ( Supplementary Fig. S3a ), and coinfected each separately with retroviruses expressing OCT4 , SOX2 , KLF4 and cMyc (OSKC) in BJ fibroblasts ( Fig. 2a ). Moreover, to determine whether these effects were cell-type specific, we performed similar reprogramming experiments in HUVEC ( Supplementary Fig. S4a ). If a genetic mutation was selected for its ability to facilitate reprogramming due to a loss of protein function, it would be expected that downregulation of the mutated gene would increase reprogramming efficiency. A decrease in reprogramming efficiency was detected after downregulation of FAIM3 , SAMD3, ZNF16, MARCKSL1, NRP1, TRAF6, GSG1 and HK1 , whereas no significant changes were detected after the downregulation of all but one of the assayed genes, POLR1C ( Fig. 2a , Supplementary Fig. 4a , Supplementary Fig. S4b ). Interestingly, we observed that downregulation of POLR1C in BJ fibroblasts, but not in HUVEC, resulted in an increased reprogramming efficiency. However, it is unclear whether the specific reprogramming-associated mutation in POLR1C would result in the same phenotype. Overall, our data suggest that protein-coding point mutations generally do not prime rare cells for reprogramming through the loss-of-function mechanism. Figure 2: Evaluation of the functional effect of hiPSC mutations on reprogramming efficiency. ( a , b ) Human BJ fibroblasts were infected with retroviruses encoding OSKC, and either lentiviruses encoding shRNAs against the indicated proteins ( a ) or retroviruses encoding the wild type or mutated proteins ( b ). Relative reprogramming efficiencies (evaluated as percentage of Nanog + colonies) are shown as fold change normalized to the averaged efficiency observed in ( a ) pLVTHM or ( b ) pMX–GFP-infected fibroblasts. In a , lentiviruses encoding shRNAs against CycE1 or p53 were used as controls of reduced or increased reprogramming efficiency, respectively. In b , retroviruses encoding p16 or the pair CDK4/CycD1 were used as controls of reduced or increased reprogramming efficiency, respectively. For a , 20,000 infected cells were plated when shRNAs against POLR1C and p53 were used, and 70,000 infected cells were plated under all other conditions. For b , a total of 25,000 infected cells were plated under all conditions. Two independent experiments with two biological replicates were carried out. All error bars depict the s.d. Full size image Next, we performed ‘gain-of-function’ reprogramming experiments to determine whether expression of the mutated form facilitated cell reprogramming. To this end, we designed a panel of retroviruses encoding both the wt form and the corresponding mutated form found in hiPSCs of each specific gene (see specific mutations in Supplementary Table S2 ; Supplementary Fig. S3b ), and coexpressed them with OSKC in BJ fibroblasts and HUVECs ( Fig. 2b , Supplementary Fig. S4c ). If a mutation were selected during reprogramming due to a gain-of-function, it would be expected that expression of the mutated form would increase the reprogramming efficiency. We observed that only the expression of HK1 slightly increased reprogramming efficiency ( Fig. 2b and Supplementary Fig. S4c ). Importantly, we did not observe significant differences in reprogramming efficiency between cells overexpressing the mutated forms and cells overexpressing their respective wt forms ( Fig. 2b ), indicating that the presence of the mutated protein does not increase reprogramming efficiency. We have previously shown that both the mut allele and the wt allele are expressed in hiPSCs ( Fig. 1 ). However, it is possible that a similar level of expression of the wt and mut protein forms is necessary in order for the mutation to influence reprogramming efficiency in a gain-of-function manner. To clarify this, we performed a reprogramming experiment where OSKC were coexpressed together with a similar total amount of retrovirus encoding either only the wild type form or both the wt and mut forms of a mutated gene in an equal ratio (1:1). Using this strategy, we were able to compare the reprogramming efficiency of cells overexpressing wt and mutated protein (wt/mut) in equal amounts with that of cells overexpressing wt protein alone (wt/wt). Interestingly, we did not observe any difference in reprogramming efficiency between cells overexpressing the wt/wt and wt/mut proteins ( Fig. 3a ). Finally, we investigated whether silencing of retroviral transgenes during reprogramming could mask a gain-of-function effect of the mutated genes at a later stage of reprogramming. We thus analysed the reprogramming efficiency of cells infected with retroviruses expressing OSKC, the wt or mutated forms of the genes evaluated in this study, and a red fluorescent protein (RFP) reporter gene to monitor transgene silencing. Reprogramming efficiency was evaluated based on the number of Tra-1-60 + /RFP + colonies present at day 14. These colonies represent putative bona-fide hiPSC colonies, as they express the stem cell marker Tra-1-60 but lack silencing of the exogenous transgenes. Thus, we only considered reprogramming events where transgene expression was still active. Importantly, we did not observe differences in reprogramming efficiency between cells overexpressing the mutated forms and cells overexpressing their respective wt forms ( Fig. 3b ). Furthermore, we also evaluated reprogramming efficiency in the same experiment at day 14 by analysing the number of Tra-1-60 + /RFP − colonies (evaluating putative bona-fide hiPSC colonies where transgene silencing occurred), and obtained a similar result (data not shown). Overall, these data suggest that most of these mutated genes do not facilitate reprogramming through a gain-of-function or loss-of-function mechanism. 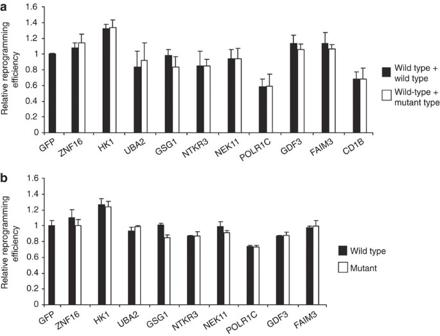Figure 3: Retroviral silencing or wild-type/mutant gene ratio do not alter reprogramming efficiency. (a) HUVEC cells were infected with retroviruses encoding OSKC, and a similar total amount of retroviruses encoding only the wild-type form or both, the wild-type and mutant forms of the protein in an equal proportion. (b) HUVEC cells were infected with retroviruses encoding OSKC, RFP and the wild-type or mutated forms of the genes indicated. Relative reprogramming efficiencies (evaluated as percentage of Tra-1-60+colonies) are shown as fold change normalized to the averaged efficiency observed in green fluorescent protein-infected HUVECs. Ten thousand infected cells were plated under all the conditions. Two independent experiments with two biological replicates were carried out. All error bars depict the s.d. Figure 3: Retroviral silencing or wild-type/mutant gene ratio do not alter reprogramming efficiency. ( a ) HUVEC cells were infected with retroviruses encoding OSKC, and a similar total amount of retroviruses encoding only the wild-type form or both, the wild-type and mutant forms of the protein in an equal proportion. ( b ) HUVEC cells were infected with retroviruses encoding OSKC, RFP and the wild-type or mutated forms of the genes indicated. Relative reprogramming efficiencies (evaluated as percentage of Tra-1-60 + colonies) are shown as fold change normalized to the averaged efficiency observed in green fluorescent protein-infected HUVECs. Ten thousand infected cells were plated under all the conditions. Two independent experiments with two biological replicates were carried out. All error bars depict the s.d. Full size image Our work demonstrates that hiPSCs contain protein-coding mutations independent of the cell type of origin (as we analysed hiPSC lines derived from five tissue types). Moreover, we determined that reprogramming efficiency, and therefore the level of selection pressure which could allow the fixation of advantageous mutations, did not to have a measurable effect on the hiPSC mutational load. Although the functional consequences of individual protein-coding mutations detected in hiPSCs remain to be characterized, these alterations could potentially contribute to the functional differences observed between hiPSC lines [15] , [16] , [17] . Two independent groups have recently reported the whole-genome sequencing of human and murine iPSC lines and their corresponding somatic cell lines [18] , [19] . They identified hundreds of single-nucleotide variants (SNVs) in non-coding regions and an average of 6–12 SNVs in coding regions [18] , [19] , which is consistent with our results [6] . Importantly, their data suggest that much of the genetic variation in iPSC clones pre-exists in the somatic population of origin and is fixed as a consequence of cloning individual cells during iPSC generation [18] , [19] . Although these reports supported previous observations [6] , they did not investigate whether identified mutations contribute functionally to facilitate the acquisition of pluripotency during reprogramming. In this work, we show evidence suggesting that most reprogramming-associated point mutations do not provide a detectible selective advantage towards a reprogrammed state. As inhibiting wt POLR1C expression had a positive impact on reprogramming efficiency, we cannot rule out a potential role of the mutation found in POLR1C in facilitating reprogramming. If this is the case, the fact that downregulation of POLR1C increases reprogramming efficiency in fibroblasts, but not in HUVECs, could indicate the existence of tissue-specific mutations affecting reprogramming efficiency, as POLR1C P278R was found in one hiPSC line derived from human fibroblasts. Although it remains possible that untested mutated genes or a combination of mutations in a certain cellular context could have a role, the findings that only one gene ( NTRK3 ) was found mutated in 2 out of 30 independent hiPSC lines, that mutated genes do not cluster in a specific functional pathway that could explain their selection during the reprogramming process, and that non-coding regions showed a similar mutational load, indicate that reprogramming-associated mutations seem to occur through a random process without selection and/or are initially present in the somatic population of origin [18] , [19] . It has been suggested that genomic alterations (that is, duplications, deletions and mutations) are selected for during reprogramming, yet this has not been demonstrated [6] , [7] , [8] , [9] , [10] , [11] . In contrast to well-established recurrent genomic aberrations (for example, chromosome 12 duplications) present in hESC or hiPSC lines that are functionally selected upon prolonged culture [8] , our results suggest that reprogramming-associated point mutations generally do not affect reprogramming efficiency although there could be exceptions. To our knowledge, the data provided herein provides for the first time a functional analysis of the role of specific genomic alterations (that is, point mutations in coding regions) on the reprogramming process and have potential implications for the future of the hiPSC field in regenerative medicine. Cell culture The hiPSC lines ASThiPS4F4, ASThiPS4F5, HUVhiPS4F1, HUVhiPS4F3, FhiPS4F7, NSChiPS2F and FhiPS3F1 were already described [6] , [20] , [21] , [22] , and obtained from existing cultures. The hiPSC lines MSChiPS4F4, MSChiPS4F8 and KhiPS4F8 show all the requirements (morphology, pluripotent gene expression, normal karyotype and in vivo differentiation by teratoma formation) to define them as hiPSC cell lines. Derived hiPSCs were cultured as described [23] . 293T cells and BJ human fibroblasts (ATCC, CRL-2522) were cultured in DMEM (Invitrogen) supplemented with 10% FBS and 0.1 mM non-essential amino acids. HUVEC cells were obtained from Lonza (C-2519A) and grown with EGM-2 media (Lonza) as recommended. MSCs were kindly provided by Cécile Volle (Sanofi-Aventis) and grown in α-MEM (Invitrogen) containing 10% FBS (Hyclone), penicillin/streptomycin, sodium pyruvate, non-essential amino acids, and L-glutamine (all from Invitrogen). Human keratinocytes were obtained and cultured as previously described [24] . hiPSC generation To generate hiPSCs (KhiPS4F8, MSChiPS4F4 and MSChiPS4) or to evaluate reprogramming efficiency, experiments were performed as described with minor modifications [23] . Briefly, BJ fibroblasts, keratinocytes, MSCs or HUVEC cells were infected with an equal ratio of retroviruses or retroviruses plus lentiviruses by spinfection of the cells at 1850, r.p.m. for 1 h at room temperature in the presence of polybrene (4 μg ml −1 ). After one (in case of the HUVEC cells), two (in case of the BJs fibroblasts or keratinocytes) or three (in case of the MSCs) viral infections viral infections, cells were trypsinized and transferred onto fresh irradiated mouse embryonic or human fibroblasts where correspond. One day after, cells were switched to hES cell medium (DMEM/F12 or KO-DMEM (Invitrogen) supplemented with 20% knockout serum replacement (Invitrogen), 1 mM L -glutamine, 0.1 mM non-essential amino acids, 55 μM β-mercaptoethanol and 10 ng ml −1 bFGF (Joint Protein Central)). Depending on the cell type of origin, colonies were stained for Nanog expression at day 18 (in the case of HUVEC-derived hiPS cells) or 24 (in the case of BJ fibroblasts-derived hiPS cells) or isolated to establish cell lines. To calculate the efficiency of reprogramming, we plated the same number of infected HUVEC or BJ fibroblasts cells on irradiated mouse embryonic fibroblasts after the infection and the relative percentage of Nanog + colonies to the value of the number of colonies generated with HUVEC or BJ fibroblasts cells infected with pLVTHM lentiviruses or green fluorescent protein-expressing retroviruses correspondingly is shown. Plasmid construction The reprogramming plasmids pMX- OCT4 , pMX- SOX2 , pMX- KLF4 , pMX- cMyc together with pLVTHM were obtained from Addgene (plasmids 17217, 17218, 17219, 17220 and 12247, respectively). For the construction of pMX- NTRK3 , pMX- FAIM3 , pMX- POLR1C , pMX- GDF3 and pMX- HK1 (fragment corresponding to the nucleotides 277–2753), specific coding region sequences were amplified by PCR from Human ORFeome library plasmids containing the corresponding cDNAs. cDNA fragments were digested with adequate restriction enzymes, purified and subcloned into linearized pMX plasmid. For the construction of pMX- CCKBR , pMX- SAMD3 , pMX- UBA2 , pMX- TRAF6 , pMX- MARCKSL1 , pMX- CD1B , pMX- GSG1 , pMX- NRP1 , pMX- NEK11 , pMX- CTSL1 , pMX- ASB3 and pMX- ZNF16 , specific pDONR223 plasmids from Human ORFeome library containing the corresponding cDNAs were used to transfer the cDNAs to the vector pMX-GW (Addgene, 18656). The transfer was achieved by using the Gateway LR Clonase enzyme mix (Invitrogen). The plasmids pMX- p16 , pMX- CDK4 , pMX- CycD1 , pLVTHM- CycE and pLVTHM- p53 were generated as described [23] , [25] . The plasmid pMX-RFP was kindly provided by Dr Guanghui Liu (Gene Expression Laboratory, The SALK Insitute, La Jolla, CA). For the introduction of specific point mutations in the coding sequences of the above genes (see Supplementary Table S2 for specific mutations) the QuickChange Site-Directed Mutagenesis kit was used (Stratagene; see Supplementary Table S3 for specific primers). For the generation of plasmids encoding shRNAs against the genes used in this study, specific oligos (see Supplementary Table S3 for specific primers) were annealed, phosphorylated with T4 kinase and ligated into MluI/ClaI-linearized pLTVHM plasmid. The design of three different pairs of shRNAs was carried out using the SFold software ( http://sfold.wadsworth.org/ ), and knockdown efficiency was assayed in 293T cells. The most efficient pairs of shRNAs were assayed in HUVEC or BJ fibroblasts cell ( Supplementary Fig. S1a ) and used in the corresponding experiments. All constructs generated were subjected to direct sequencing to rule out the presence of mutations. Retroviral and lentiviral production Moloney-based retroviral vectors (pMX and derived) and second-generation lentiviral vectors (pLVTHM and derived) were cotransfected with packaging plasmids to generate viral particles in 293T cells using Lipofectamine (Invitrogen) as previously described [23] . Immunostaining Imnunofluorescence analysis for the detection of pluripotent markers in hiPSCs or for the detection of differentiation-associated markers in teratomas were performed as described [22] . Immunohistochemical/immunoflorescence detection of Nanog or Tra-1-60 was performed as described [23] . RNA isolation and real-time PCR analysis Total RNA was isolated using Trizol Reagent (Invitrogen) according to the manufacturer’s recommendations. cDNA was synthesized using the SuperScript II Reverse Transcriptase kit for RT–PCR (Invitrogen) or the RT Supermix M-MuLV kit (BioPioneer). Real-time PCR was performed using the SYBR-Green PCR Master mix (Applied Biosystems) in the ViiA 7 Real Time PCR System (Applied Biosystems). Glyceraldehyde 3-phosphate dehydrogenase expression was used to normalize values of gene expression and data is shown as fold change relative to the value of the sample control. All the samples were done in triplicate. Primers used for real-time PCR experiments are listed in Supplementary Table S3 . Whole-genome library construction Library construction was performed as previously described [6] , [26] . Briefly, for each sample, roughly 1.5–3 μg of genomic DNA (in 100 μl volumes) was sheared with a Covaris AFA. The fragmented genomic DNA was end repaired, A-tailed and ligated to sequencing adaptors, with a purification step between each process. The purified ligated products were then amplified by PCR to generate whole-genome libraries. In-solution hybridization capture with DNA baits Liquid exome capture was performed as previously described [6] . Consensus sequence generation and variant calling Variant calling was performed as previously described [6] . Briefly, reads obtained from the Illumina Genome Analyzer were post-processed and quality filtered using GERALD, mapped to the genome using BWA, downsampled using Picard and used to generate a consensus sequence for each sample using GATK. The consensus sequences were then compared with find candidate novel mutations in hiPSCs [6] . Sites where each hiPSC line showed heterozygous SNPs not observed in the progenitor line were considered as candidate mutations if no allelic content was present in the somatic progenitor and if the candidate mutation had not previously been observed in other samples or the dbSNP database. Sanger validation of candidate mutations Genomic DNA of both the hiPSC line and its somatic progenitor (6 ng each) was amplified in separate 50 μl PCR reactions with 100 nM of specifically designed forward and reverse primers around the mutation site (primers available under request) and 25 μl of Taq 2 × master mix (NEB) at 94 °C for 2 min, followed by 35 cycles of 94 °C for 30 s, 57 °C for 30 s and 72 °C for 30 s, and final extension at 72 °C for 3 min. The PCR products were then purified with Qiagen Qiaquick columns, and 10 ng of purified DNA was pre-mixed with 25 pmol of the forward primer for Sanger sequencing at Genewiz Inc. Statistical analysis/TiGER database To check for enrichment of reprogramming-associated mutations in genes that are expressed in a tissue-specific manner, the fraction of UniGene IDs corresponding to mutated genes called as ‘tissue-specific’ in the TiGER database was identified as 49/132 (37%). As 6,699/19,526 (34%) of the genes annotated in the TiGER database are considered to be tissue specific, a χ 2 -test with one degree of freedom can be used to test for equivalency of distribution. The obtained χ 2 value is 0.460, indicating that the fraction of mutated hiPSC genes that are tissue specific is not significantly different than that found in a random sample of genes ( P =0.4975). Reprogramming-associated mutations therefore do not appear to be enriched in tissue-specific genes. Statistical analysis/active and inactive chromatin states To check for enrichment of reprogramming-associated mutations in active or inactive chromatin, we utilized a χ 2 -test with three degrees of freedom to test for equivalency of distribution. We identified the chromatin state of each mutated gene using previously published data [13] . These data divided each gene into one of four categories: no trimethylation, H3K4 trimethylation, H3K27 trimethylation, or both. We compared the distribution of mutated genes across each of these four categories with the expected distribution for all genes in three cell types: fibroblasts, ESCs and iPSCs [13] . The obtained χ 2 values were 1.03 ( P =0.79), 3.78 ( P =0.29) and 6.97 ( P =0.07), respectively, indicating that the distribution of mutated hiPSC genes in each chromatin region is not significantly different than expected by random chance ( α =0.01). Reprogramming-associated mutations therefore do not appear to be enriched in active or inactive chromatin states. Non-coding versus coding mutations To compare the mutation rates per base pair in coding and non-coding regions of the genome, variant calling was performed as above on non-coding regions of the genome surviving library enrichment in eight hiPSC lines and their progenitor lines. The mutation rate per base pair was then estimated by dividing the number of candidate coding and non-coding mutations by the number of exomic and non-coding base pairs covered. The average coding and non-coding mutation rates were compared. How to cite this article: Ruiz, S. et al. Analysis of protein-coding mutations in hiPSCs and their possible role during somatic cell reprogramming. Nat. Commun. 4:1382 doi: 10.1038/ncomms2381 (2013).